The genome ofMesobuthus martensiireveals a unique adaptation model of arthropods Representing a basal branch of arachnids, scorpions are known as ‘living fossils’ that maintain an ancient anatomy and are adapted to have survived extreme climate changes. Here we report the genome sequence of Mesobuthus martensii , containing 32,016 protein-coding genes, the most among sequenced arthropods. Although M. martensii appears to evolve conservatively, it has a greater gene family turnover than the insects that have undergone diverse morphological and physiological changes, suggesting the decoupling of the molecular and morphological evolution in scorpions. Underlying the long-term adaptation of scorpions is the expansion of the gene families enriched in basic metabolic pathways, signalling pathways, neurotoxins and cytochrome P450, and the different dynamics of expansion between the shared and the scorpion lineage-specific gene families. Genomic and transcriptomic analyses further illustrate the important genetic features associated with prey, nocturnal behaviour, feeding and detoxification. The M. martensii genome reveals a unique adaptation model of arthropods, offering new insights into the genetic bases of the living fossils. Arthropoda contains two lineages, the Chelicerata and the Mandibulata, which arose during the Cambrian period and radiated into millions of species of diverse shapes in over 500 million years [1] , [2] . Scorpions represent a special type of arthropod. Unlike others, they are considered ‘living fossils’, as they maintain the primary features of Paleozoic scorpions [3] , such as venom apparatus, book lung and pectine, and are well adapted to have survived extreme environmental changes. There are about 2,000 scorpion species described worldwide, which are found in all continents except Antarctica. Scorpiones is a basal lineage of Arachnida, and Arachnida forms a major branch of Chelicerata. Scorpions, therefore, occupy a key phylogenetic position in the evolution of chelicerates and arthropods. Scorpions developed a venom system as a primary weapon for capturing prey and defending against predators. The structure of their venom-secreting gland was first observed in the oldest scorpion fossils dated from the Late Silurian period ( Proscorpius osborni , 418 million years B.P.) [4] . Evolving over the past 400 million years, scorpion venom contains diverse types of neurotoxins, which are low-molecular-weight polypeptides, acting to block or modulate ion channels critical for the transmission of nerve signals across synapses [5] . Scorpion envenomation is a significant threat to public health in many regions around the world, with the number of scorpion stings estimated to be 1.2 million annually, resulting in more than 3,200 deaths [6] . Scorpions are an indispensable part of the ecological food chain and they help to maintain a balance among various populations in an ecosystem. They primarily feed on insects, and also arachnids, myriapods, gastropods and small vertebrates. Scorpions are typically nocturnal animals, hiding in the day and foraging at night. Their hunting is aided by trichobothria (vibration-sensing hairs on the pedipals) and a vision system comprising of two median and two to five pairs of lateral eyes. It was also shown that scorpion tails were photosensitive [7] , [8] , [9] , which could help detect the movement of a prey under dim light. Interestingly, most scorpion species fluoresce under ultraviolet light [10] . To explore the genetic features underlying the long-term survival and adaptive model of scorpions, we report the genome sequence of Mesobuthus martensii , the most populous species from eastern Asian countries. M. martensii is a raw material for traditional Chinese medicine and is used to treat diseases like rheumatoid arthritis, apoplexy, epilepsy and chronic pain. Its neurotoxins, the active ingredient in their venom, represent a rich resource for drug development in modern medicine [11] , [12] . The availability of the M. martensii genome expands the gene repertoire of chelicerates and provides a toolkit for undertaking genetics and systems biology approaches to study this evolutionarily important creature. Genome features and transcriptome analysis Using flow cytometry analysis, we estimated the M. martensii genome to be 1,323.73±39.12 Mb in size ( Supplementary Fig. S1 and Supplementary Table S1 ). We sequence the M. martensii genome using a whole-genome shotgun approach and generate raw sequence reads of approximately 248 × coverage ( Supplementary Table S2 ). A draft genome (v1.0) of 1,128.5 Mb is assembled, having a scaffold N50 length of 223.6 kb, and a contig N50 length of 43.1 kb ( Supplementary Table S3 ). Non-gap sequences occupy 1,078.5 Mb (95.6%), and simple sequence repeats (SSR) total 34 Mb (3.0%) ( Supplementary Fig. S2 and Supplementary Table S4 ). Transposable elements (TEs) add up to 35 Mb, roughly 3.1% of the assembled genome. The most abundant types of TEs are Gypsy, hAT and Mariner-like elements ( Supplementary Table S5 ). The number of TEs is believed to be underestimated, as we sample raw sequence reads and find roughly 13.0% of them mapped to TEs ( Supplementary Note 1 ), suggesting that TEs are highly redundant in the M. martensii genome and a significant portion of them might have not been incorporated into the assembly. Single-nucleotide polymorphisms and small indels for the sequenced diploid are predicted to be ~3.24 kb −1 ( Supplementary Table S6 ). To help annotate the M. martensii genome, we perform deep transcriptome analyses on the samples of mixed tissues and samples of venom tissues, for which 5.53 and 4.52 Gb RNA-seq data are acquired, respectively. Excluding transposase-like genes, there are a minimum of 32,016 protein-coding genes predicted for the M. martensii genome ( Supplementary Figs S3–S5 and Supplementary Table S7 ). The quality of the genome assembly and the 32,016 gene models are assessed and supported by many lines of evidence ( Supplementary Note 1 ). First, 29,837 protein-coding genes (93.2%) are supported by the RNA-seq data ( Supplementary Fig. S6 ), and 18,961 (59.2%) show similarity to proteins from species other than scorpions. In comparison, Daphnia pulex [13] and Tetranychus urticae [14] have 64.0% and 60.8% of proteins having homologues from other species, respectively. Second, 14,785 (46.2%) are validated with the recently published transcriptome data from Centruroides noxius (a scorpion from different genus) [15] . Third, we find that 457 of the 458 CEGMA core genes [16] are identified in the gene models, and 440 (96.1%) are supported by the RNA-seq data. Fourth, the possibility of counting allelic variants as paralogues (so inflating the gene count) is also very low. It is estimated that totally 0.89% of paralogues from all gene families have synonymous distances ≤0.01 (used as an allelic variant cutoff) to other paralogues within their corresponding family. Furthermore, pseudogenes are estimated to be no more than 4.3% of all protein-coding genes, which is in line with those of other studies [13] . And lastly, gene duplications in the M. martensii lineage occur in an extended time frame at a rate comparable to that of D. pulex (details in ‘Expansion of shared and lineage-specific gene families’). The GC contents in M. martensii are 42.7% for the coding regions and 29.6% for the whole genome. M. martensii has a median gene size of ~6.7 kb (ORF plus introns) with a mean exon number at 3.9 per gene ( Supplementary Table S7 ) and an average intron size of 2.12 kb ( Supplementary Fig. S7 ), forming a clear contrast to T. urticae (a mite) with 3.8 exons per gene but an intron size of 120 bp on average. T. urticae has a genome size of 89.6 Mb with 18,414 predicted genes. Compared with T. urticae , we also observe a dramatic increase in total gene number but a reduced gene density in M. martensii. There are 205 and 35.8 genes per Mb for T. urticae and M. martensii , respectively. In addition, 6,139 (19.2%) protein-coding genes from M. martensii are found to have alternatively spliced forms ( Supplementary Table S8 ). The occurrence of alternative splicing represents a mechanism for M. martensii to diversify gene functions. In combination with its large gene contents, M. martensii has a more complex and dynamically regulated functional genome. Comparative genomics and evolution Phylogenetic trees are built using both maximum likelihood and neighbour joint with 220 orthologues from the CEGMA core genes [16] that are present in each of the 17 species, including two arachnids M. martensii and T. urticae , eleven insects Drosophila melanogaster, Acyrthosiphon pisum, Apis mellifera, Bombyx mori, Camponotus floridanus, Anopheles gambiae, Aedes aegypti, Culex pipiens, Pediculus humanus , Tribolium castaneum and Nasonia vitripennis , one branchiopod D. pulex, one nematode Caenorhabditis elegans , one ascidiace Ciona intestinalis and one mammal Homo sapiens . Both trees are similar in topology when rooted using the two vertebrates as the outgroup ( Supplementary Fig. S8 and Supplementary Table S9 ). M. martensii is grouped together with T. urticae , forming the arachnid clade. D. pulex, a crustacean, is placed as the sister taxon to Hexapoda to the exclusion of Chelicerata. Comparing gene content reveals M. martensii shares 3,338 (56.1%) gene families with T. urticae , 3,717 (62.5%) with D. pulex and 3,512 (59.1%) with D. melanogaster , whereas 2,747 gene families are common to the four arthropods ( Fig. 1a ). Surprisingly, M. martensii shares more families with D. pulex than with its closer relative, T. urticae . This can be explained by the loss of more common genes in the T. urticae lineage than in the D. pulex lineage. 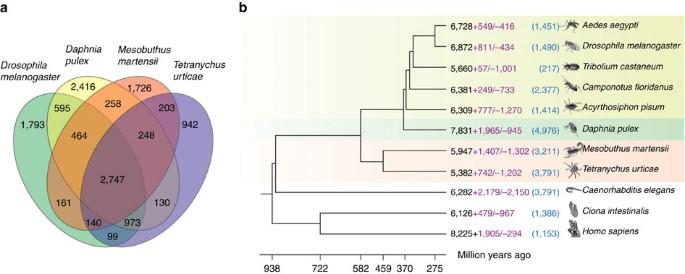Figure 1: Comparative analyses of theM. martensiigenome. (a) Venn diagram of shared and unique gene families betweenD. melanogaster,D. pulex,M. martensiiandT. urticae. Clusters of orthologous and paralogous gene families are identified by OrthoMCL53. (b) Gene gain-and-loss analysis of species across arthropods, nematode and chordates. The branching and the divergence times between lineages are derived from the TimeTree database54, and are marked with a scale in million years at the bottom. For each species, total gene families (black), the numbers of gene family gain (+) and loss (−) (purple), and orphan genes (blue) are indicated (Supplementary Note 2). Figure 1: Comparative analyses of the M. martensii genome. ( a ) Venn diagram of shared and unique gene families between D. melanogaster , D. pulex , M. martensii and T. urticae . Clusters of orthologous and paralogous gene families are identified by OrthoMCL [53] . ( b ) Gene gain-and-loss analysis of species across arthropods, nematode and chordates. The branching and the divergence times between lineages are derived from the TimeTree database [54] , and are marked with a scale in million years at the bottom. For each species, total gene families (black), the numbers of gene family gain (+) and loss (−) (purple), and orphan genes (blue) are indicated ( Supplementary Note 2 ). Full size image A gene gain-and-loss analysis is performed on representative species across the phylogeny ( Fig. 1b ). There is a gain of 1,407 gene families ( Mesobuthus lineage-specific family) and a loss of 1,302 in the M. martensii lineage. Mesobuthus lineage-specific gene families account for 23.7% (1,407/5,947) of all families, and notably 62.1% (874/1,407) of them have unknown function ( Supplementary Note 2 ). When adding the orphan genes (3,211), there are a total of 18,091 Mesobuthus -specific genes. Thus, the accumulation of Mesobuthus -specific genes contributes to more than half (56.5%) of the M. martensii genetic pool. Comparing the gene family turnover (gene family gain and loss combined) among the involved arthropods ( Fig. 1b ) shows that the Mesobuthus lineage has a greater gene family turnover (2,709) than the insect lineages ( Aedes, Drosophila, Tribolium, Camponotus and Acyrthosiphon ) having undergone diverse changes in physiology and morphology. Although scorpions have apparently evolved more conservatively compared with the insects, the result illustrates a startling contrast on the genomics level. The decoupling of the molecular and morphological evolution suggests that scorpions represent a unique adaptation model in arthropods, different from that of the insects. Expansion of shared and lineage-specific gene families The elevation of gene count in M. martensii appears to result from the expansion of both the shared and the lineage-specific gene families. There are 496 gene families that are significantly expanded ( z -score>2) in M. martensii ( Supplementary Note 3 ). In addition, there are 63 gene families with more than 20 members from M. martensii but shared by fewer than three species (so z -scores are not computed for them). In contrast, T. urticae and D. pulex have 172 and 269 significantly expanded ( z score≥2) gene families, respectively ( Supplementary Table S10 ). The expanded families in M. martensii are enriched in pathways such as basic metabolic pathways (purine, pyrimidine, amino acid, fatty acid, and so on), signalling and stress response pathways (MAPK, GnRH, calcium, chemokine, and so on), cholinergic synapse and P450 families ( Supplementary Fig. S9 and Supplementary Table S11 ). How the expanded gene families were preserved and contributed to the long-term survival of scorpions just began coming to light. Gene duplication events in the evolution of M. martensii lineage are estimated with the synonymous distances (Ks) from all paralogue pairs. Their distributions suggest that gene duplication events took place in an extended time frame in the Mesobuthus lineage, and there is no evidence to suggest the occurrence of whole-genome duplication ( Fig. 2a ). M. martensii, T. urticae and D. pulex appear to undergo gene duplications in a similar course in each lineage. M. martensii genes duplicate at a rate of ~68% that of D. pulex , and ~7 times as high as that of T. urticae ( Fig. 2a ). When plotted separately, the shared families from M. martensii are shown to begin expansion early in the lineage at a relatively steady rate ( Fig. 2b ). They concentrate on pathways of nutrition intakes, metabolisms and signal transductions, that is, salivary secretion, protein digestion and absorption, drug metabolism (CYPs), ABC transporters, Notch signalling, chemokine signalling and so on. ( Supplementary Note 3 ). In contrast, the expansion of the Mesobuthus lineage-specific families accelerated more recently and most families (88%) have unknown function. The driving force behind such distinct dynamics in the expansion of the different gene families is poorly understood, and remains one of the most interesting subjects for future study. However, the distributions of family member sizes are comparable between the shared and the Mesobuthus lineage-specific gene families ( Fig. 2c ). 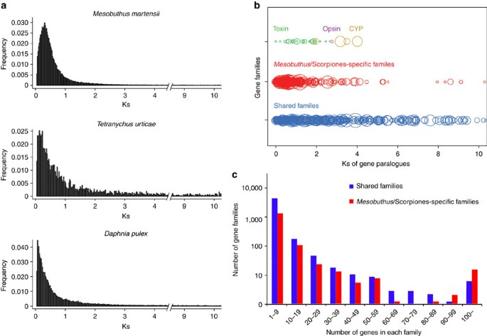Figure 2: Gene family expansion and evolution. (a) Frequency of pair-wise genetic divergence at silent sites (Ks) among gene paralogues fromM.martensii,T.urticaeandD.pulex. The Ks values for gene pairs with >70 aligned amino acids and identity >70% are calculated using codeml PAML package50. (b) Ks distribution of the shared,Mesobuthuslineage-specific, and three functional gene families. Each circle represents a gene family, and the size of a circle signifies the member count of a corresponding family. (c) Distribution of the shared andMesobuthuslineage-specific gene family sizes. Figure 2: Gene family expansion and evolution. ( a ) Frequency of pair-wise genetic divergence at silent sites (Ks) among gene paralogues from M . martensii , T . urticae and D . pulex . The Ks values for gene pairs with >70 aligned amino acids and identity >70% are calculated using codeml PAML package [50] . ( b ) Ks distribution of the shared, Mesobuthus lineage-specific, and three functional gene families. Each circle represents a gene family, and the size of a circle signifies the member count of a corresponding family. ( c ) Distribution of the shared and Mesobuthus lineage-specific gene family sizes. Full size image Genetic diversity of venom neurotoxins and their receptors The genes of venom neurotoxins form the most expanded families in M. martensii . Their structure and diversity have not been systematically characterized at the genome scale before this study. A total of 116 neurotoxin genes are located in the M. martensii genome ( Supplementary Fig. S10 and Supplementary Table S12 ), including 61 NaTx (toxins for sodium channels), 46 KTx (toxins for potassium channels), 5 ClTx (toxins for chloride channels) and 4 CaTx (toxins for ryanodine receptors) genes. Among them, 45 encoded previously unknown neurotoxins and 109 are expressed in the venomous gland ( Supplementary Figs S11–S14 ). Fifty-one neurotoxin genes are found to arrange in clusters on 17 scaffolds ( Fig. 3a and Supplementary Table S13 ). Within each cluster are tandemly duplicated genes of the same family, sharing similar gene structure ( Supplementary Figs S15 and S16 ). Notably similar gene features are also found in the defensin gene loci in M. martensii ( Fig. 3a , Supplementary Figs S17 and S18 and Supplementary Tables S13 and S14 ), exhibiting an evolutionary trajectory parallel to that of neurotoxin genes. 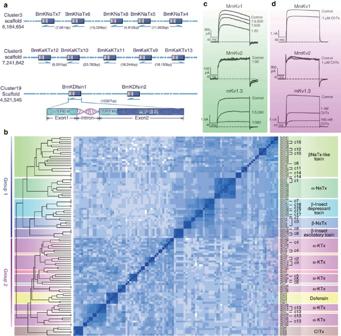Figure 3: Diversification of neurotoxin and its receptor genes fromM. martensii. (a) Organization and structure of the representative neurotoxin and defensin gene clusters fromM.martensii. Scaffolds 6184654, 7241642 and 4521545 are illustrated. SPER, signal peptide encoding region. MPER, mature peptide encoding region. BmKNaTx,M.martensiisodium channel toxin gene. BmKaKTx,M.martensiialpha potassium channel toxin gene. BmKDfsin,M.martensiidefensin gene. (b) A heat-map representation of the hierarchical clustering analysis17of neurotoxins and defensins fromM. martensii. The analysis is performed using sequence similarity scores from pairwise alignments of neurotoxins and defensins. The dendrogram illustrates the relationship between classes of neurotoxins and defensins, revealing the association of sequence homology groups to the pharmacological classes. c1-17, cluster 1-17. βNaTx-like toxin, beta-type sodium channel neurotoxin-like. α-NaTx, alpha-type sodium channel neurotoxin. β-insect depressant toxin, beta-type depressant insect neurotoxin. β-NaTx, beta-type sodium channel neurotoxin. β-insect excitatory toxin, beta-type excitatory insect neurotoxin. α-KTx, alpha-type potassium channel neurotoxin. ClTx, neurotoxin for chloride channel. (c) Resistance of theM. martensiiK+channels, MmKv1 and MmKv2, to scorpion venom. Effects of theM. martensiivenom on MmKv1, MmKv2 and mKv1.3 (murine K+channel) are shown with 1:50, 1:500 and 1:5,000 dilutions. The inhibitory effect of the venom on MmKv1 is about 100-fold smaller than that on mKv1.3.M. martensiivenom has no inhibition on MmKv2. (d) Resistance of theM. martensiiK+channels, MmKv1 and MmKv2, to the scorpion neurotoxin ChTX. 1 μM ChTX inhibits 20% MmKv1 activity and has no inhibition on MmKv2, whereas 1 nM ChTX inhibits 60% mKv1.3 (murine K+channel) activity. The inhibitory effect of ChTX on MmKv1 is 1,000-fold smaller than that on mKv1.3. Figure 3: Diversification of neurotoxin and its receptor genes from M. martensii . ( a ) Organization and structure of the representative neurotoxin and defensin gene clusters from M . martensii . Scaffolds 6184654, 7241642 and 4521545 are illustrated. SPER, signal peptide encoding region. MPER, mature peptide encoding region. BmKNaTx, M . martensii sodium channel toxin gene. BmKaKTx, M . martensii alpha potassium channel toxin gene. BmKDfsin, M . martensii defensin gene. ( b ) A heat-map representation of the hierarchical clustering analysis [17] of neurotoxins and defensins from M. martensii . The analysis is performed using sequence similarity scores from pairwise alignments of neurotoxins and defensins. The dendrogram illustrates the relationship between classes of neurotoxins and defensins, revealing the association of sequence homology groups to the pharmacological classes. c1-17, cluster 1-17. βNaTx-like toxin, beta-type sodium channel neurotoxin-like. α-NaTx, alpha-type sodium channel neurotoxin. β-insect depressant toxin, beta-type depressant insect neurotoxin. β-NaTx, beta-type sodium channel neurotoxin. β-insect excitatory toxin, beta-type excitatory insect neurotoxin. α-KTx, alpha-type potassium channel neurotoxin. ClTx, neurotoxin for chloride channel. ( c ) Resistance of the M. martensii K + channels, MmKv1 and MmKv2, to scorpion venom. Effects of the M. martensii venom on MmKv1, MmKv2 and mKv1.3 (murine K + channel) are shown with 1:50, 1:500 and 1:5,000 dilutions. The inhibitory effect of the venom on MmKv1 is about 100-fold smaller than that on mKv1.3. M. martensii venom has no inhibition on MmKv2. ( d ) Resistance of the M. martensii K + channels, MmKv1 and MmKv2, to the scorpion neurotoxin ChTX. 1 μM ChTX inhibits 20% MmKv1 activity and has no inhibition on MmKv2, whereas 1 nM ChTX inhibits 60% mKv1.3 (murine K + channel) activity. The inhibitory effect of ChTX on MmKv1 is 1,000-fold smaller than that on mKv1.3. Full size image We search the NCBI nr database for homologues of scorpion neurotoxins and find none from species other than scorpions, suggesting that scorpion neurotoxin genes evolved independently within the lineage. Hierarchical clustering [17] is used to investigate the origin and evolutionary relationship of neurotoxins and defensins from M. martensii . Two major groups are formed: group 1 comprising NaTx genes and group 2 comprising KTx, ClTx and defensin genes ( Fig. 3b ). Remarkably, these results not only point to the monophyly of the neurotoxin and defensin genes in M. martensii , but also implicate a structure−function relationship by the association of sequence homology groups with the pharmacological classes of action. Although we cannot completely rule out the formation of such relationship by convergence, it is most likely that NaTx diverged first from the common ancestor of KTx, ClTx and defensin genes that subsequently diversified and formed separate families. Possessing the most potent weaponry of diverse neurotoxins, scorpions were reported to be immune to their venom toxins [18] , which raises the hypothesis that scorpion ion channels adapt to their own neurotoxins. We prove and quantify the resistance of M. martensii to its venom by injecting fresh venom into its body in repeated experiments ( Supplementary Note 4 and Supplementary Tables S15 and S16 ). We then look at two new genes encoding K + channels from M. martensii , MmKv1 and MmKv2, which are voltage-dependent channels with six membrane-spanning domains containing the positively charged S4 segment and the ion selectivity filter ( Supplementary Fig. S19 ). In both MmKv1 and MmKv2, one of the critical residues in the filter region becomes basic residue, in reference to the murine homologue, mKv1.3. Changes in this region were previously proposed to confer immunity to scorpion toxins on K + channels [19] , [20] . MmKv1 and MmKv2 are expressed in HEK293 cells to form functional K + channels, and are found to be insensitive to scorpion venom and to charybdotoxin (ChTx), a classic scorpion neurotoxin [21] , [22] ( Fig. 3c,d and Supplementary Fig. S20 ). The finding first reveals a possible mechanism underlying scorpions’ resistance to their neurotoxins, implying the co-evolution of ion channels with neurotoxin genes in M. martensii . Genetic basis for photosensor function in scorpion tail Previous behavioural and electrophysiological experiments indicate that scorpions can respond to light signals through their tails [7] , [8] , [9] . To understand the genetic basis for light sensitivity in the tail, we focus on genes involved in photoreception and light signal transduction ( Fig. 4a ). Three homologues of opsin genes, Mmopsin1, Mmopsin2 and Mmopsin3, are identified in the M. martensii genome ( Supplementary Note 5 and Supplementary Fig. S21 ) and their expressions are revealed by transcriptome data and quantified by quantitative PCR (qPCR). Whereas all three are expressed in the prosoma (head containing eyes), only Mmopsin3 is found in the tail ( Fig. 4b ). Furthermore, the 20 visual signal transduction genes are found to transcribe in the tail ( Supplementary Fig. S22 and Supplementary Tables S17 and S18 ), illustrating the formation of the complete molecular pathway for light sensitivity in scorpion tail. Lacking the specialized optical structure of an eye, the scorpion tail represents a primitive light-sensing organ that receives light signals by epithelium and generates electrophysiological reactions through contacted nerve dendrites before being transmitted to the brain ( Supplementary Fig. S23 ). Such a primitive photosensor can be traced to other invertebrates, such as, hydra [23] , sea urchin [24] and bivalves [25] . 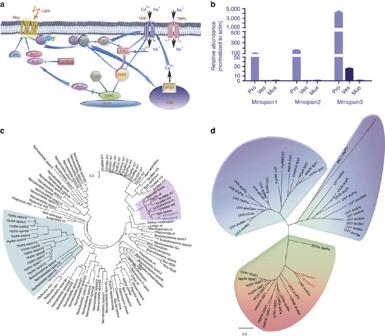Figure 4: Molecular basis for photosensor function in the scorpion tail. (a) Pathway of light-sensing signal transduction in the scorpion tail. The signal transduction network is modelled after that ofD. melanogaster55. The involved signalling molecules are listed inSupplementary Tables S17 and S18. (b) Quantitative expression analysis of opsin genes, Mmopsin1, Mmopsin2 and Mmopsin3, inM.martensii. pro, prosoma; ves, vesicle or venom gland; mus, muscle from chelas and metasomal segments I-V. Data are expressed as the mean±s.d. from three replicates. (c) Phylogenetic relationships among opsins. The phylogenetic tree is constructed with the conserved sequences among opsin proteins, using ML method (MEGA5)56(Supplementary Note 5). Mmopsin1 and Mmopsin2 are grouped with those from insects, whereas Mmopsin3 is closely related to opsins from generaHydra,BranchiostomaandNematostella. (d) Spectrum bias of theM. martensiiopsins. The phylogenetic tree is constructed as inc. Mmopsin3 is a member of short-wavelength (ultraviolet to blue) opsins, but Mmopsin1 and Mmopsin2 belong to long-wavelength opsins. Figure 4: Molecular basis for photosensor function in the scorpion tail. ( a ) Pathway of light-sensing signal transduction in the scorpion tail. The signal transduction network is modelled after that of D. melanogaster [55] . The involved signalling molecules are listed in Supplementary Tables S17 and S18 . ( b ) Quantitative expression analysis of opsin genes, Mmopsin1, Mmopsin2 and Mmopsin3, in M . martensii . pro, prosoma; ves, vesicle or venom gland; mus, muscle from chelas and metasomal segments I-V. Data are expressed as the mean±s.d. from three replicates. ( c ) Phylogenetic relationships among opsins. The phylogenetic tree is constructed with the conserved sequences among opsin proteins, using ML method (MEGA5) [56] ( Supplementary Note 5 ). Mmopsin1 and Mmopsin2 are grouped with those from insects, whereas Mmopsin3 is closely related to opsins from genera Hydra , Branchiostoma and Nematostella . ( d ) Spectrum bias of the M. martensii opsins. The phylogenetic tree is constructed as in c . Mmopsin3 is a member of short-wavelength (ultraviolet to blue) opsins, but Mmopsin1 and Mmopsin2 belong to long-wavelength opsins. Full size image Scorpion eyes and tails appear to diverge functionally in photo-sensing. The eyes utilize all three opsins in visual formation, but the tail is only capable of working with Mmopsin3 ( Supplementary Table S19 ). A phylogenetic analysis indicates that Mmopsin3 forms a clade with the opsins from Hydra magnipapillata , which is traced to approximately 600 million years ago and known to express numerous opsins in its nerve system and cephalon [23] , whereas Mmopsin1 and Mmopsin2 are close to eye-related rhodopsins from insects and vertebrates ( Fig. 4c , and Supplementary Table S20 ). These data suggest that Mmopsin3 represents an ancient form of opsins utilized broadly by primitive non-vision systems before the morphogenesis of eyes later in evolution. Mmopsin3 also appears to be a member of the short-wave-sensitive (ultraviolet to blue) opsin family, whereas both Mmopsin1 and Mmopsin2 belong to the long-wave-sensitive family ( Fig. 4d and Supplementary Table S20 ). The spectrum bias of Mmopsin3 agrees with the previously documented scorpion behaviour under different wavelengths [8] , [26] . The photosensor function of scorpion tail may have an important role in support of their habitant behaviours. The non-visual photosensor mechanism, first revealed in an animal, raises the questions about the broad use of such function by other arthropods and invertebrates, and the general role that a non-visual photosensor has in the adaptation and evolution of arthropods and invertebrates. P450 genes in detoxification and hormone biosynthesis In animals, CYPs participate in the biosynthesis and metabolism of sterols, hormones and fatty acids for maintaining homeostasis, and the detoxification of xenobiotics (such as phytotoxin) from foods and environments [27] , [28] . One hundred and sixty CYP genes were identified in the M. martensii genome, which belong to the CYP2, CYP3, CYP4 and mitochondrial clans ( Supplementary Note 6 and Supplementary Tables S21 and S22 ). In comparison, D. pulex and T. urticae have 75 and 86 CYP genes [14] , [29] , respectively. The pattern of major CYP family expansion in M. martensii (CYP3 and CYP4 clans) is different from that in D. pulex (CYP2 and CYP4 clans) and that in T. urticae (the intronless CYP2 clan). Notably, CYP3A (67) and CYP4V (42) form major gene clusters on the M. martensii genome, driven by gene duplications at the CYP loci ( Supplementary Table S23 ). CYP3 and CYP4 are important to metabolize xenobiotics and fatty acids in animals [30] , [31] . M. martensii feeds on herbivorous insects or the herbivorous larva of predatory insects, and is accustomed to phytotoxins. Thus, the active enzyme systems of CYP3 and CYP4 families are critical for their survival in hazardous environments. CYPs may have a role in the fluorescence by M. martensii under ultraviolet light ( Fig. 5a,b ). 4-Methyl-7-hydroxy-coumarin was reported as one of the fluorescent compounds found in 11 scorpion species [10] . We detect coumarin and its two derivatives, 7-hydroxy-coumarin and 4-methyl-7-hydroxy-coumarin, in the ethanol extract from the M. martensii cuticle ( Fig. 5c and Supplementary Figs S24−S26 ). Interestingly, the two compounds glow equally well when exposed to ultraviolet light ( Supplementary Fig. S27 ). The result identifies 7-hydroxy-coumarin as a new fluorescent agent from scorpions. As 7-hydroxy-coumarin does not form from the degradation of 4-methyl-7-hydroxy-coumarin ( Supplementary Fig. S28 ), it is suggested that 7-hydroxy-coumarin is synthesized from coumarin in vivo. Supporting the hypothesized pathway, a homologue (MMa36879) of CYP2A6, reportedly converting coumarin to 7-hydroxy-coumarin in mammals [32] , is identified in M. martensii . Taken together, it is likely that scorpions obtain coumarin (a phytotoxin) from herbivorous insects, and subsequently detoxify it by converting to derivatives that are fluorescent. 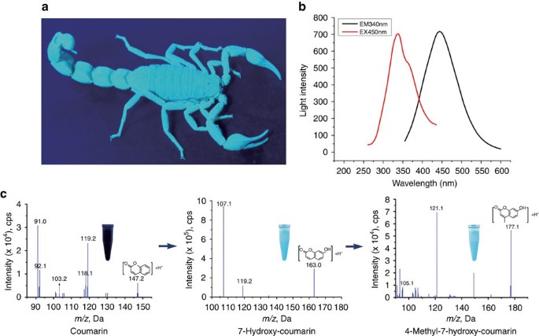Figure 5: Detoxification of coumarin and synthesis of fluorescent compounds inM. martensii. (a) A fluorescentM. martensiiunder an ultraviolet lamp. (b) Fluorescence spectra of the ethanol extract fromM. martensii. Excitation spectra (red) are obtained by monitoring the emission of light at 450 nm (EX450nm), and emission spectra (blue) by monitoring the emission flowing excitation at 340 nm (EM340nm). (c) Identification of coumarin and its derivatives fromM. martensiiby CAD mass spectrum. Coumarin, 7-hydroxy-coumarin and 4-methyl-7-hydroxy-coumarin are detected from the extract of theM. martensiicuticle by LC-ESI-MS/MS (MRM mode) chromatogram (Supplementary Note 6). Tubes containing chemical standards, coumarin, 7-hydroxy-coumarin and 4-methyl-7-hydroxy-coumarin are shown. The latter two emit blue fluorescence under ultraviolet light. Figure 5: Detoxification of coumarin and synthesis of fluorescent compounds in M. martensii . ( a ) A fluorescent M. martensii under an ultraviolet lamp. ( b ) Fluorescence spectra of the ethanol extract from M. martensii . Excitation spectra (red) are obtained by monitoring the emission of light at 450 nm (EX450nm), and emission spectra (blue) by monitoring the emission flowing excitation at 340 nm (EM340nm). ( c ) Identification of coumarin and its derivatives from M. martensii by CAD mass spectrum. Coumarin, 7-hydroxy-coumarin and 4-methyl-7-hydroxy-coumarin are detected from the extract of the M. martensii cuticle by LC-ESI-MS/MS (MRM mode) chromatogram ( Supplementary Note 6 ). Tubes containing chemical standards, coumarin, 7-hydroxy-coumarin and 4-methyl-7-hydroxy-coumarin are shown. The latter two emit blue fluorescence under ultraviolet light. Full size image CYP genes are involved in the synthesis of juvenile and moulting hormones, which control metamorphosis and reproduction, and regulate development and life cycle in arthropods. CYP15A1 is a critical enzyme that converts methyl farnesoate to juvenile hormone III through epoxidation ( Supplementary Fig. S29 ). Like in T. urticae with missing CYP15A1 gene, the juvenile hormone III is predicted to be not synthesized in M. martensii , and instead, methyl farnesoate is produced as the choice for juvenile hormone ( Supplementary Fig. S29 and Supplementary Table S24 ). However, different from T. urticae that synthesizes ecdysteroid 25-deoxy-20-hydroxyecdysone (ponasterone A) as the moulting hormone [14] , M. martensii has both CYP306A1 and CYP18A1 genes, and thus it produces the normal ecdysone 20E as the moulting hormone. As the first complete scorpion genome and the second in Chelicerata, M. martensii is found to have the most protein-coding genes among sequenced arthropods. The M. martensii genome expands the genetic repertoire of arthropods into a previously unknown territory, which will aid further studies on the comparative genomics and evolution of arthropods. Considered a special type of arthropods, extant scorpions have preserved the primary features of Paleozoic ancestors from the Cambrian age. However, the Mesobuthus lineage is found to have a gene family turnover at a level significantly greater than the insects, challenging the common wisdom that scorpions apparently evolved more conservatively as ‘living fossils’. The data reveal the decoupling of the molecular and morphological evolution in scorpions, a phenomenon documented for the first time in an arthropod. Underlying the molecular evolution of the M. martensii genome are the expansion of the gene families enriched in the basic metabolic pathways, signalling and stress response pathways, neurotoxins, and cytochrome P450 families of enzymes, and the different dynamics of expansion between the shared and the scorpion lineage-specific gene families. Genomic and transcriptomic analyses further illustrate the genetic features in M. martensii associated with the prey, nocturnal behaviour, feeding and detoxification, which are believed to be important to its long-term adaptation. These include the diversification of neurotoxins and their receptor genes, the expression of light-signal transduction genes enabling photosensor in the tail and the expansion of P450 families involved in detoxification and hormone biosynthesis. Taken together, these analyses on the scorpion genome reveal a unique adaptation model distinctive to other sequenced arthropods. The genomics study on M. martensii yields new insights into the evolution of arthropods, and raises some new questions as well, for example, the cause of the accelerating expansion of the scorpion lineage-specific gene families, and the general roles of the non-visual photosensor in the evolution of arthropods. This work builds a foundation for future exploration of these intriguing creatures, and also provides a valuable resource for addressing those fundamentally important questions. Sample preparation M . martensii individuals were collected from the Fu-niu Mountains, Xichuan County (33.13−33.17°N, 111.48−111.52°E), Henan Province, China. They were examined and manipulated under a Motic K700 stereoscopic microscope. An adult M. martensii male was selected for the extraction of DNA from muscle tissues of the pedipalp and metasoma (to minimize microbial contamination) for genomic sequencing. The tissue sample was ground in liquid nitrogen, and DNA extraction was performed using TIANamp Genomic DNA Kit DP304-2 (Tiangen, China) according to the manufacturer’s protocols. The quality and quantity of the DNA sample were examined by ultraviolet absorbance and gel electrophoreses. For whole-body transcriptome sequencing, an adult male was used. It was washed three times with 95% ethanol to reduce microbial contamination from its body surface. After ethanol volatilization, the sample was ground into a fine powder in liquid nitrogen. Total RNA was prepared using the TRIZOL Reagent (Invitrogen, Carlsbad, CA, USA). Meanwhile, for transcriptome sequencing of the venom gland (telson), 30 M . martensii individuals (15 males and 15 females) were used and dissected. The tissues were mixed and total RNA was prepared as described above. RNA quantitation was performed by ultraviolet absorbance and its quality was further examined by gel electrophoreses. Genome and transcriptome sequencing A whole-genome shotgun approach was used for genome sequencing. Paired-end libraries with insert sizes of 180, 300 and 420 bp, and mate-pair libraries with circular DNA sizes of 5 and 10 Kb were constructed separately, following the manufacturer’s instructions (Illumina, San Diego, CA, USA). Sequencing was performed with the Illumina GAIIx and Hiseq2000 according to the standard Illumina protocols. Additional sequencing was performed with the 454 GS-FLX platform, using the manufacturer’s standard protocols (454 Life Sciences, Roche, Brandford, CT, USA). For transcriptome sequencing, libraries were prepared with RNA samples from the whole-body and from the mixed venom glands, following Illumina’s standard protocols. Sequencing was performed using Illumina Hiseq2000. Genome assembly and characterization The paired-end and mate-pair sequencing data from Illumina were first processed to filter out low-quality reads. Data were then screened against microbial, plasmid and organelle sequences, and contaminants removed from the subsequent assembly. The remaining sequence reads were assembled using Velvet [33] (version: 1.1.04) (details in Supplementary Note 1 ). The assembling was performed on a computing server, I950R-GP (Dawning Information Industry, Tianjin, China) with eight 2.67-GHz Intel XEONE7-8837 (96 cores) and 1024 G of memory. The generated scaffolds were gap-filled with GapCloser [34] (version: 1.12) using short sequence reads from GAIIx/Hiseq2000 and long reads from Roche 454 GS-FLX. We identified simple sequence repeats, low complexity DNA sequences and satellites from the M. martensii genome using SSRIT [35] and RepeatMasker [36] (version 3.2.9). Putative TEs in the M . martensii genome were located using BLAST [37] search against a scorpion-specific TE library constructed by homologue-based method with reference sequences from RepBase16.01 (ref. 38 ). For calling single-nucleotide polymorphisms and small indels, sequencing reads were first mapped to the draft genome using Bowtie2 (ref. 39 ), a BWT-based aligner. A heterozygous genotype would be called if the frequency of the non-consensus allele was between 20 and 80% (refs 40 , 41 ). Gene model prediction and annotation The gene models of the M. martensii genome were predicted using a comprehensive gene prediction pipeline combining ab initio modelling, homology-based modelling and EST-based modelling, involving several programs Augustus [42] (version 2.5.5), Fgenesh++ [43] , GENEID [44] (version 1.2), SNAP [45] , GlimmerHMM [46] and Gnomon ( http://www.ncbi.nlm.nih.gov/genome/guide/gnomon.shtml ). First, TEs and other sequence repeats in the genome assembly were masked before gene modelling. Then a gene prediction training set (including 876 manually curated genes) was constructed with the combined results from the self-trained prediction methods. The training set was used to optimize the parameters for a second round of gene modelling, and the results were incorporated to produce a minimum gene set of 32,016 for M. martensii . (version 1.0 gene models: http://lifecenter.sgst.cn/main/en/Scorpion-Suppl/gene-models-v1.0.gff ). The transfer RNAs and ribosomal RNAs were identified using the programs t-RNAscan SE [47] and RNAmmer [48] , respectively. Gene annotation and ontology assignment was performed with BLAST searches against the NCBI nr, Swiss-Prot and TrEMBL databases using the E -value cutoff of 1E−5. The NCBI CDD and Sanger Pfam databases were used for functional domain annotation. Genes were mapped to metabolic pathways using KAAS based on the KEGG database [49] . (Additional attributes for gene models are described in Supplementary Note 1 ). Comparative genomics and gene family expansion analyses Comparative genomics studies were performed with the 17 genomes ( Supplementary Note 2 ). Phylogenetic analyses were performed using the 220 orthologues from the CEGMA core genes. The orthologous genes from each of the 17 genomes were aligned using ClustalX (version 1.83), and phylogenetic trees were built with MEGA5 using both neighbour-joining and maximum-likelihood methods (500 replicas for the bootstrapping tests). For gene family expansion analyses, gene families were identified using orthoMCL with default parameters, with the − I parameter set to 3.0. The z -score was computed for each gene family and those with z -score ≥2 represent significantly expanded gene families ( Supplementary Note 3 ). The age of gene families was estimated with the synonymous distances (Ks, number of synonymous substitutions per synonymous site) among paralogues using the codeml program from PAML package [50] . The Ks values were corrected according to Colbourne’s protocol [13] . To investigate the differential duplicate rates among M . martensii , T . urticae and D . pulex , the number of single duplicated paralogues within the youngest cohort (Ks<0.01) was calculated. The gene birth rate of each species was estimated according to the following formula: the gene birth rate=the number of youngest single duplicate gene pairs/(the number of single copy genes+number of single duplicate gene pairs) [13] . Resistance of M. martensii to its own venom toxins Acute poisoning experiments were carried out with the scorpion M. martensii and the cockroach Blaptica dubia . The scorpions and cockroaches were randomly grouped and injected with variable doses of fresh venom or with water as control ( Supplementary Note 4 ). The number and course of animal death were recorded. Statistical analysis of the data was carried out using Microsoft Excel (version 2007) to determine median lethal dose (LD50). Measurement data were represented as the mean±s.d., and the Student’s t -test was used for two-group comparisons. Electrophysiological recording The cDNAs encoding MmKv1 and MmKv2 were transiently transfected into HEK293 cells (China Center for Type Culture Collection, China) using the FuGene Transfection Reagent (Roche Diagnostics, Switzerland). The ion channel currents were measured 1–3 days after the transfections. To measure the Kv channel currents, the internal pipette and external solutions were prepared according to the reported procedures [51] , [52] . The voltage-gated K + channel currents were elicited by 200-ms depolarizing voltage steps from the holding potential of −80 to +50 mV. The formation of functional K + channels in MmKv1- or MmKv2-transfected cells was verified by blocking their currents with TEA (Sigma, USA), XE-991 (Tocris Bioscience, USA), or scorpion toxin ChTX (Alomone, Jerusalem, Israel). As a comparison, the mouse K + channel mKv1.3 was transiently transfected into HEK293 cells and its pharmacological activity was detected with the addition of M. martensii venom or ChTX. qPCR analysis The qPCR analysis was performed to detect the expression of the 14 photo-transduction genes in three separate tissues: prosoma (head with eyes), vesicle (tail or telson) and muscle ( Supplementary Note 5 ). The qPCR primers ( Supplementary Table S19 ) were synthesized at the Tsingke Biotechnology Limited Company (Wuhan, China). PCR amplification was conducted in an ABI 7500HT real-time PCR system using the following program: 3 min of 94 °C, 32 cycles of 94 °C for 30 s, 55 °C for 30 s, 72 °C for 45 s and a final extension at 72 °C for 10 min. Identification of coumarin and its derivatives We extracted fluorescent compounds from M. martensii according to Frost et al. [10] The chemical standards, coumarin, 7-hydroxy-coumarin and 4-methyl-7-hydroxy-coumarin were purchased from Sigma (USA) as the reference control. Reverse-phase high-performance liquid chromatography (HPLC) with a C18 column (10 mm × 250 mm, 5 μm, DaLian Elite, China) was performed to collect fractions containing coumarin, 7-hydroxy-coumarin or 4-methyl-7-hydroxy-coumarin. Analysis of fluorescent compounds was performed on the HPLC-electrospray ionization-tandem mass spectrometry (ESI-MS/MS) system consisting of an AB 3200 QTRAP liquid chromatography (LC)-MS/MS (Applied Biosystems) with an ESI source (Turbo Ionspray) and a Shimadzu LC-20 AD HPLC (Tokyo, Japan) system. The Shimadzu LC-20 AD HPLC contained a Shim-pack VP-ODS (150 mm × 2.0 mm; internal diameter, 5 mm) column. Data acquisition and processing were performed using Analyst 1.5 software (Applied Biosystems). Accession codes: The genome assembly has been deposited in GenBank under BioProject PRJNA171479. The genome and related annotation files are accessible at http://lifecenter.sgst.cn/main/en/scorpion.jsp . How to cite this article: Cao, Z. et al. The genome of Mesobuthus martensii reveals a unique adaptation model of arthropods. Nat. Commun. 4:2602 doi: 10.1038/ncomms3602 (2013).